Interface control of the magnetic chirality in CoFeB/MgO heterostructures with heavy-metal underlayers Recent advances in the understanding of spin orbital effects in ultrathin magnetic heterostructures have opened new paradigms to control magnetic moments electrically. The Dzyaloshinskii–Moriya interaction (DMI) is said to play a key role in forming a Néel-type domain wall that can be driven by the spin Hall torque. Here we show that the strength and sign of the DMI can be changed by modifying the adjacent heavy-metal underlayer (X) in perpendicularly magnetized X/CoFeB/MgO heterostructures. The sense of rotation of a domain wall spiral is reversed when the underlayer is changed from Hf, Ta to W and the strength of DMI varies as the filling of 5 d orbitals, or the electronegativity, of the heavy-metal layer changes. The DMI can even be tuned by adding nitrogen to the underlayer, thus allowing interface engineering of the magnetic texture in ultrathin magnetic heterostructures. Understanding the underlying physics of current-driven domain wall motion is essential in developing advanced storage class memory devices [1] . Conventionally, domain walls move along the electron flow (against the current) when driven by spin transfer torque [2] , [3] . Recently, a number of experiments [4] , [5] , [6] , [7] , [8] , [9] , [10] have shown that the domain walls can instead move against the electron flow in magnetic heterostructures consisting of an ultrathin magnetic layer sandwiched between heavy-metal layers or a heavy-metal layer and an insulating oxide layer. To describe this effect, the ‘spin Hall torque [11] ’ has been considered as a possible driving force of the domain walls. Spin Hall torque occurs when spin current, generated in the heavy-metal layer via the spin Hall effect [12] , diffuses into the magnetic layer and exerts spin transfer torque on the magnetization. If a domain wall is present, the spin Hall torque can move the wall only if it forms a Néel-like structure [13] , [14] . To move sequences of domain walls with current via the spin Hall torque in the same direction, the Néel wall has to alternate its magnetization direction between neighbouring domain walls. This requires formation of a ‘domain wall spiral [15] ’, which can be generated in systems with large spin orbit coupling and broken inversion symmetry via the Dzyaloshinskii–Moriya interaction [16] , [17] (DMI). In the above model [9] , [10] , [13] , [14] , the direction to which a domain wall moves with current is determined by the signs of the spin Hall angle of the heavy-metal layer and the DMI. The sign of the spin Hall angle is determined by element-specific spin orbit coupling constant of the heavy-metal layer; for example, it is opposite [9] , [11] , [18] for Pt and Ta. For the DMI, the sign depends on the spin orbit coupling as well as the structural symmetry of the magnetic layer [16] , [17] . For example, in three-dimensional bulk-like systems, the sense of rotation of the magnetic structure, that is, the ‘chirality’, can either follow or be opposite to the crystallographic chirality in Mn- and Fe-based non-centrosymmetric B20 structures [19] , respectively, indicating the difference in the spin orbit coupling of the Mn- and Fe-based systems. The magnetic chirality at surfaces has been studied intensively using spin polarized scanning tunnelling microscopy [20] , [21] . Here the surface atomic configuration plays an important role in setting the chirality. The origin of the DMI at interfaces is more difficult to treat as the structural symmetry determination is non-trivial. It has been reported that DMI changes its sign depending on the order of the film stack [10] , [22] , which is consistent with the three-site indirect exchange mechanism [23] proposed previously. Recent experiments [9] have indicated that for a given magnetic layer (CoFe), the sign of the DMI is the same even when the adjacent non-magnetic layer (Pt or Ta) has the opposite sign of the spin orbit coupling constant. Here we show that the size and sign of the DMI can be changed for a given magnetic layer when the neighbouring heavy-metal layer is modified. In X/CoFeB/MgO heterostructures with different heavy-metal underlayers (X=Hf, Ta, TaN and W), we find that the domain wall moves along or against the electron flow depending on the underlayer material. The sign of the spin Hall angle is the same for all underlayers, indicating that the sign of bulk spin orbit coupling constant of X is the same. In contrast, the magnetic chirality of the domain walls is found to be reversed when the underlayer material is varied from Hf, Ta to W. From these results, we infer that the strength of the DMI depends on the filling of 5 d orbtials, or the electronegativity, of the neighbouring layer (X). Heavy-metal-dependent domain wall velocity Magnetic heterostructures consisting of a film stack substrate/ d nm X/1nm CoFeB/2nm MgO|/1nm Ta are studied (see Methods for details). The heavy-metal underlayer X is Hf, Ta, TaN and W. The composition of TaN is close to ~50 at% nitrogen. The magnetic easy axis points out of plane owing to the perpendicular magnetic anisotropy developed at the CoFeB/MgO interface [24] . Optical lithography is used to pattern wires and Hall bars from the films. An optical microscopy image of the wire along with schematic illustration of the experimental setup is shown in Fig. 1a,b . Variable amplitude voltage pulses (duration is 20–100 ns) are fed into the wire from a pulse generator. Positive voltage pulse supplies current into the wire that flows along the + x direction. A domain wall is nucleated [25] by applying a voltage pulse above a critical amplitude which depends on the film stack. Kerr microscopy is used to acquire magnetic images of the sample. Current-driven domain wall velocity is estimated by dividing the distance the wall travelled, obtained from the Kerr images, by the total pulse length. 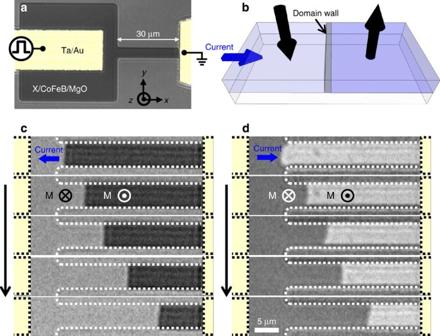Figure 1: Schematic of the experimental setup and magneto-optical Kerr images illustrating current-induced domain wall motion. (a) Optical microscopy image of the wire used to study current-induced domain wall motion. Ta/Au electrodes are indicated by the yellow-coloured region. A pulse generator is connected to one of the Ta/Au electrodes, as schematically shown. (b) Illustration of the experimental setup. The thick black arrows indicate magnetization of the CoFeB layer. (c,d) Typical Kerr images showing current-induced domain wall motion along (c) and against (d) the electron flow for wires with different underlayers: (c) ~0.5-nm thick Ta underlayer, (d) ~3.6-nm thick TaN(Q: 0.7%) underlayer. Domain walls inc,dare both ↓↑ walls. Between images: ~−40 V, 100-ns long pulses are applied 12 times forcand ~28 V, 100-ns long pulses are applied 20 times ford. Figure 1: Schematic of the experimental setup and magneto-optical Kerr images illustrating current-induced domain wall motion. ( a ) Optical microscopy image of the wire used to study current-induced domain wall motion. Ta/Au electrodes are indicated by the yellow-coloured region. A pulse generator is connected to one of the Ta/Au electrodes, as schematically shown. ( b ) Illustration of the experimental setup. The thick black arrows indicate magnetization of the CoFeB layer. ( c , d ) Typical Kerr images showing current-induced domain wall motion along ( c ) and against ( d ) the electron flow for wires with different underlayers: ( c ) ~0.5-nm thick Ta underlayer, ( d ) ~3.6-nm thick TaN( Q : 0.7%) underlayer. Domain walls in c , d are both ↓↑ walls. Between images: ~−40 V, 100-ns long pulses are applied 12 times for c and ~28 V, 100-ns long pulses are applied 20 times for d . Full size image Exemplary Kerr microscopy images are shown in Fig. 1c,d when negative and positive voltage pulses are applied to devices made of Ta and TaN underlayer films respectively. The domain wall moves along the electron flow for the former, whereas it moves against the electron flow for the latter. Note that the domain walls shown in Fig. 1c,d correspond to same domain configuration (↓↑ walls). Depending on the thickness and the dielectric constant of each layer including the 100-nm thick SiO 2 , the Kerr contrast can change (see Methods for details). Domain wall velocity as a function of the voltage pulse amplitude is summarized in Fig. 2 (and Supplementary Fig. 1 ). Positive velocity corresponds to a domain wall moving toward the + x direction. For Hf and Ta underlayer films, the domain wall always moves along the electron flow. This also applies for the thin TaN underlayer films. However, the domain wall moves against the electron flow for the thicker TaN underlayer films and for all of the W underlayer films. Note that the applicable pulse amplitude is limited by the voltage at which current-induced domain wall nucleation occurs. 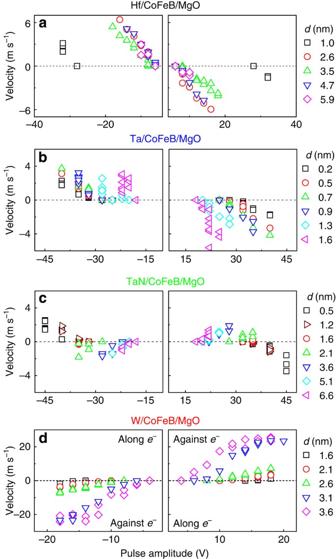Figure 2: Pulse amplitude dependence of domain wall velocity. (a–d) Domain wall velocity as a function of pulse amplitude plotted for magnetic heterostructures with four different underlayers. The underlayer is (a) Hf, (b) Ta, (c) TaN(Q: 0.7%) and (d) W. The direction to which the wall moves is indicated in each panel ofd:e−corresponds to electron flow. Average domain wall velocity is obtained by moving a domain wall across ~30-μm long wires. This process is repeated multiple times for a given pulse amplitude: all results are shown by the symbols. Figure 2: Pulse amplitude dependence of domain wall velocity. ( a – d ) Domain wall velocity as a function of pulse amplitude plotted for magnetic heterostructures with four different underlayers. The underlayer is ( a ) Hf, ( b ) Ta, ( c ) TaN( Q : 0.7%) and ( d ) W. The direction to which the wall moves is indicated in each panel of d : e − corresponds to electron flow. Average domain wall velocity is obtained by moving a domain wall across ~30-μm long wires. This process is repeated multiple times for a given pulse amplitude: all results are shown by the symbols. Full size image Threshold current density to trigger domain wall motion The threshold current density needed to move a domain wall is plotted in Fig. 3a–h (and Supplementary Fig. 2 ), open symbols. Current density that flows in the CoFeB layer ( J C CoFeB ) and the underlayer ( J C Under ) are calculated and shown in the top (a–d) and bottom (e–h) panels, respectively. The solid symbols in Fig. 3 represent the maximum current density applied to each device; beyond this current density, we find evidence of current-induced domain nucleation. Thus, the range of current density applied to each device to study current-induced domain wall motion is limited between the values shown by the open and solid symbols. In almost all cases, the threshold current density (both J C CoFeB and J C Under ) decreases as d is increased. 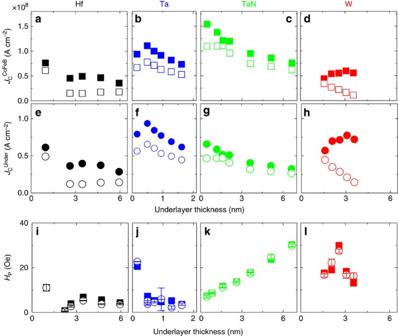Figure 3: Threshold current density and propagation field required to move domain walls. (a–h) The threshold current density needed to move a domain wall is shown by the open symbols. The solid symbols represent the maximum current density applied to each device; beyond this current density, current-induced domain nucleation occurs. The current density that flows in the CoFeB layer (JCCoFeB) and the underlayer (JCUnder) is shown in the top (a–d) and bottom (e–h) panels, respectively. The current density in each layer is estimated by taking into account the difference in the film thickness and resistivity of the two layers. (i–l) Propagation fieldHPplotted as a function of the underlayer thickness. Solid and open symbols represent positive and negativeHP, respectively: absolute values are shown. The measurement is repeated five times for each device and field direction: error bars correspond to the standard deviation of the measurements. The underlayer is (a,e,i) Hf, (b,f,j) Ta (c,g,k) TaN(Q: 0.7%) and (d,h,l) W. Figure 3: Threshold current density and propagation field required to move domain walls. ( a – h ) The threshold current density needed to move a domain wall is shown by the open symbols. The solid symbols represent the maximum current density applied to each device; beyond this current density, current-induced domain nucleation occurs. The current density that flows in the CoFeB layer ( J C CoFeB ) and the underlayer ( J C Under ) is shown in the top ( a – d ) and bottom ( e – h ) panels, respectively. The current density in each layer is estimated by taking into account the difference in the film thickness and resistivity of the two layers. ( i – l ) Propagation field H P plotted as a function of the underlayer thickness. Solid and open symbols represent positive and negative H P , respectively: absolute values are shown. The measurement is repeated five times for each device and field direction: error bars correspond to the standard deviation of the measurements. The underlayer is ( a , e , i ) Hf, ( b , f , j ) Ta ( c , g , k ) TaN( Q : 0.7%) and ( d , h , l ) W. Full size image The out-of-plane field needed to move a domain wall, that is, the propagation field ( H P ), is plotted in Fig. 3i–l . H P represents the strength of average domain wall pinning along the wire. The change in H P is mostly correlated with the magnetic anisotropy of the films: films with larger K EFF display larger H P . The origin of the linear d dependence of H P for the TaN films is not well understood. H P is generally small and is below ~30 Oe for all devices. To examine the underlying mechanism of current-driven domain wall motion, we study the size and sign of the current-induced effective magnetic field in a Hall bar patterned on the same substrate using the adiabatic (low frequency) harmonic Hall voltage measurements [26] , [27] , [28] (see Methods for details). 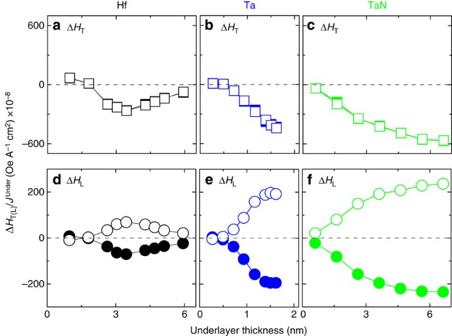Figure 4: Current-induced effective field versus the underlayer thickness. Transverse (a–c) and longitudinal (d–f) components of the current-induced effective field, ΔHT/JUnderand ΔHL/JUnder, respectively, are plotted as a function of the underlayer thickness for film stacks with different underlayers: (a,d) Hf, (b,e) Ta and (c,f) TaN(Q: 0.7%). The effective field is normalized by the current density (JUnder) that flows into the underlayer. The solid and open symbols correspond to the effective field when the magnetization of the CoFeB layer is pointing along +zand –z, respectively. Figure 4 (and Supplementary Fig. 3 ) shows the underlayer thickness dependence of the effective field components directed transverse to (Δ H T , Fig. 4a–c ) and along (Δ H L , Fig. 4d–f ) the current flow direction. Δ H T(L) is normalized by the current density flowing through the underlayer ( J Under ). Measurements are performed with an average current density being smaller than ~2 × 10 7 A cm −2 . For the W underlayer films, we find that the harmonic Hall measurements do not provide accurate estimates of the effective field ( Supplementary Note 1 ). The d dependence of the longitudinal effective field Δ H L / J Under , whose direction depends on the magnetization direction and corresponds to the damping-like spin transfer torque [29] , [30] , is similar among the film structures studied here: Δ H L / J Under increases in magnitude with increasing d and saturates at a certain d (the origin of the drop at large d for the Hf underlayer films is not clear). If the effective field originates from the spin Hall torque [11] , these results show that the sign of the spin Hall angle is the same for Hf, Ta and TaN underlayer films, since Δ H L / J Under points along the same direction for a given magnetization direction. For the W underlayer films, we find that the sign of the spin Hall angle is consistent with previous reports [18] , [31] and is the same with the other heavy metal layers used here from switching phase diagram measurements [32] ( Supplementary Note 1 ). The transverse component (Δ H T / J Under ), which does not depend on the magnetization direction and thus is considered similar to the field-like spin transfer torque [33] , also shows similar underlayer thickness dependence with that of Δ H L / J Under . With regard to spin Hall torque-induced domain wall motion, it is predominantly the longitudinal component that drives a Néel wall [13] , [14] . Figure 4: Current-induced effective field versus the underlayer thickness. Transverse ( a – c ) and longitudinal ( d – f ) components of the current-induced effective field, Δ H T / J Under and Δ H L / J Under , respectively, are plotted as a function of the underlayer thickness for film stacks with different underlayers: ( a , d ) Hf, ( b , e ) Ta and ( c , f ) TaN( Q : 0.7%). The effective field is normalized by the current density ( J Under ) that flows into the underlayer. The solid and open symbols correspond to the effective field when the magnetization of the CoFeB layer is pointing along + z and – z , respectively. Full size image Determination of the chirality of the domain wall spiral As the sign of the spin Hall angle is the same for all film structures, we infer that the DMI is varying when the underlayer is changed. In out-of-plane magnetized systems, the preferred domain wall configuration is the Bloch type for the wire dimension used here: a Néel wall is only stable for narrow wires (typically below ~100 nm) where shape anisotropy starts to dominate [3] . However, the DMI can promote a Néel-type wall with a fixed chirality. This interaction can be modelled as an additional offset field ( H DM ) applied along the wire’s long axis for a given domain wall [9] , [10] , [13] . The offset field changes its direction depending on whether the magnetization of the neighbouring domain points ↑↓ or ↓↑, thus forming a domain wall spiral [15] . We thereby study the wall velocity as a function of the in-plane magnetic field directed along the wire’s long axis to probe H DM . 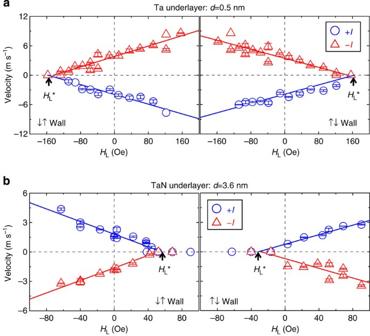Figure 5: Determination of the longitudinal compensation fieldHL*. (a,b) Domain wall velocity plotted as a function of the longitudinal fieldHL(directed along the current flow) for two different film stacks: (a) ~0.5-nm thick Ta underlayer and (b) ~3.6-nm thick TaN(Q: 0.7%) underlayer. Blue circles and red triangles indicate the wall velocity when positive and negative voltage pulses are applied, respectively. The velocity is obtained by fitting the domain wall position versus cumulated pulse length with a linear function, the error bars show the standard error of the linear fitting. Left (right) panel shows results for ↓↑ (↑↓) wall. Solid lines are linear fit to the data to obtain the compensation fieldHL*. Pulse amplitude is ~±40 V foraand ~±28 V forb. Figure 5a,b show representative results of the wall velocity versus the in-plane longitudinal field ( H L ) for two different devices in which the domain wall moves in opposite directions when driven by current. The velocity scales almost linearly with H L in all cases. At zero H L , both ↑↓ or ↓↑ walls move in the same direction for a given film structure. However, the longitudinal field at which the velocity becomes zero (that is, the compensation field defined as H L * hereafter) is different depending on the domain configuration (↑↓ or ↓↑ walls). For example, H L * is positive (negative) for a ↑↓ (↓↑) wall when the wall moves along the electron flow ( Fig. 5a ). This indicates that there is a negative (positive) offset field ( H DM ) associated with the ↑↓ (↓↑) wall. The direction of this offset field reverses when the wall moves against the electron flow ( Fig. 5b ). These results imply that the domain wall spiral possess a left-handed chirality (↑←↓ or ↓→↑) for the walls moving along the electron flow and it forms a right-handed chirality (↑→↓ or ↓←↑) when the direction of the wall motion reverses. Figure 5: Determination of the longitudinal compensation field H L * . ( a , b ) Domain wall velocity plotted as a function of the longitudinal field H L (directed along the current flow) for two different film stacks: ( a ) ~0.5-nm thick Ta underlayer and ( b ) ~3.6-nm thick TaN( Q : 0.7%) underlayer. Blue circles and red triangles indicate the wall velocity when positive and negative voltage pulses are applied, respectively. The velocity is obtained by fitting the domain wall position versus cumulated pulse length with a linear function, the error bars show the standard error of the linear fitting. Left (right) panel shows results for ↓↑ (↑↓) wall. Solid lines are linear fit to the data to obtain the compensation field H L *. Pulse amplitude is ~±40 V for a and ~±28 V for b . Full size image The underlayer thickness dependence of the longitudinal compensation field H L * is plotted in Fig. 6a–d (and Supplementary Fig. 4 ). The slope of the wall velocity versus H L for each underlayer film is shown in Supplementary Fig. 5 for reference. We find a clear correlation between the direction of the wall motion (background colour-coding) and the sign of H L *. However, note that H L * does not coincide with the offset field H DM when spin transfer torque is present. 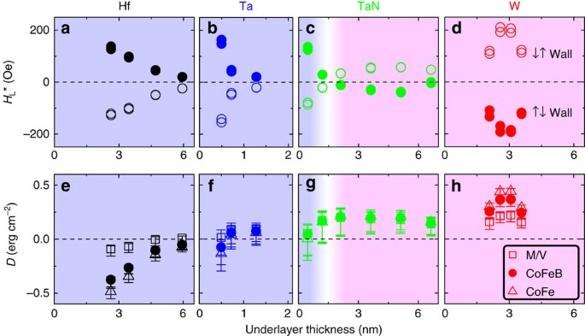Figure 6: Underlayer-dependent Dzyaloshinskii–Moriya interaction. (a–d) The compensation fieldHL*, that is, the longitudinal field (HL) at which the velocity becomes zero, plotted as a function of underlayer thickness. Solid and open symbols representHL* for ↑↓ and ↓↑ domain walls, respectively.HL* is evaluated when the wall is driven either by positive or negative voltage pulses: here, both results are shown together. The applied current density is close to values shown by the solid symbols inFig. 3a–h. (e–h) Estimated values of the Dzyaloshinskii–Moriya exchange constantDare shown when the saturation magnetization of the CoFeB layer is assumed to be the same with that ofM/V(squares) displayed inSupplementary Fig. 6(a–d), that of CoFeB (~1,500 emu cm−3, circles) and that of CoFe (~1,870 emu cm−3, triangles). The error bars show the range ofDwhen contribution from spin transfer torque is changed: lower (higher) bound of the error bars corresponds toP=0 (P=1) and the symbols assumeP=0.7. The background colour of each panel indicates the direction to which a corresponding domain wall moves; red: against the electron flow, blue: along the electron flow. The underlayer is (a,e) Hf, (b,f) Ta, (c,g) TaN(Q: 0.7%) and (d,h) W. According to the one-dimensional model of a domain wall [9] , [10] , [13] , [34] , H L * for a ↑↓ wall is expressed as ( Supplementary Note 2 ): Figure 6: Underlayer-dependent Dzyaloshinskii–Moriya interaction. ( a – d ) The compensation field H L *, that is, the longitudinal field ( H L ) at which the velocity becomes zero, plotted as a function of underlayer thickness. Solid and open symbols represent H L * for ↑↓ and ↓↑ domain walls, respectively. H L * is evaluated when the wall is driven either by positive or negative voltage pulses: here, both results are shown together. The applied current density is close to values shown by the solid symbols in Fig. 3a–h . ( e – h ) Estimated values of the Dzyaloshinskii–Moriya exchange constant D are shown when the saturation magnetization of the CoFeB layer is assumed to be the same with that of M / V (squares) displayed in Supplementary Fig. 6 (a–d), that of CoFeB (~1,500 emu cm −3 , circles) and that of CoFe (~1,870 emu cm −3 , triangles). The error bars show the range of D when contribution from spin transfer torque is changed: lower (higher) bound of the error bars corresponds to P =0 ( P =1) and the symbols assume P =0.7. The background colour of each panel indicates the direction to which a corresponding domain wall moves; red: against the electron flow, blue: along the electron flow. The underlayer is ( a , e ) Hf, ( b , f ) Ta, ( c , g ) TaN( Q : 0.7%) and ( d , h ) W. Full size image where D ( =H DM M S Δ ) is the Dzyaloshinskii–Moriya exchange constant and sgn( θ SH ) is the sign of the spin Hall angle of the heavy-metal layer. M S is the saturation magnetization, is the domain wall width parameter and P is the current spin polarization of the CoFeB layer. The unit of J CoFeB is 10 8 A cm −2 and the non-adiabatic spin torque contribution in the CoFeB layer is assumed to be negligible, as reported previously in a similar system [35] . We use the exchange stiffness constant ( A ) of the CoFeB layer obtained in a similar heterostructure [36] , although it may vary with the underlayer material/thickness. Variations of the magnetic anisotropy ( K EFF ) and M / V with d , shown in Supplementary Figs 6 and 7 , are taken into account in estimating Δ . Note that M / V shown in Supplementary Figs 6 and 7 is different from M S if a magnetic dead layer is present; M / V will underestimate M S in such case. Since the M S of the heterostructures depend on the amount of boron present in the magnetic layer, M S takes a value between that of Co 20 Fe 60 B 20 (~1,500 emu cm −3 ) and Co 25 Fe 75 (~1,870 emu cm −3 ), giving the lower and upper limits [37] . The DM exchange constant D is estimated for all devices using equation (1) ( Supplementary equation 4 shows a more general expression). An average value of H L * is obtained from ↑↓ and ↓↑ domain walls with positive and negative voltage pulses. Results are shown by the symbols in Fig. 6e–h (and Supplementary Fig. 4 ). We show in Fig. 6e–h estimates of D using the lower and upper limits of M S by the circles and triangles, respectively, and the measured M / V value by the squares. Contribution from spin transfer torque is shown by the error bars: the symbol show D when P is set to 0.7 (ref. 35 ) and the lower and upper bounds of the error bars represent D when P is 0 and 1, respectively. As evident, D varies as one moves along the 5th row of the periodic table from Hf to W: Hf underlayer films possess a negative D (left-handed magnetic chirality), whereas D is positive for TaN and W (right handed). D is small for Ta underlayer films. Since D is mostly positive for the TaN underlayer films with all thicknesses, the change in the direction of wall motion (and the sign of H L *) for the thin TaN underlayer films is due to the larger contribution from the spin transfer torque. The large reduction of D with increasing d for the Hf underlayer films indicates that perhaps the interface state is changing with the underlayer thickness: such thickness dependence is also notable for the effective field shown in Fig. 4a,d . It should be noted that when domain wall pinning is strong (that is, large H P ), H L * measured using a linear fitting to the velocity versus H L ( Fig. 5a,b ) can underestimate the offset field H DM ( Supplementary Fig. 8 and Supplementary Note 2 ). Thus the values provided in Fig. 6e–h correspond to the lower limit of | D | when the effect of pinning is concerned. The change in the size and sign of the DMI with the heavy-metal elements may be related to the change in the charge localization of the interface atoms [38] , which has been reported to change the sign of the Rashba spin splitting at metal alloy surfaces [39] . We consider that the electronegativity of the underlayer material may play an important role here. The electronegativity increases from Hf to Ta and W, similar to the trend of D . Nitrogen is also known be an element with large electronegativity, which may partly explain why D is larger for TaN than Ta. There is also a possibility that the atomic configuration, for example, local atomic arrangement and/or the amount of boron present at the interface [37] , may vary as we change the underlayer material and thus contribute to the change in D . We consider that the origin of the DMI in the heterostructures studied here may be different from that of the Pt-based systems [9] , [10] , where the induced magnetic moments in the Pt layer has been suggested [10] to be responsible for the large D . Sample preparation Films are deposited by magnetron sputtering (DC and RF) on Si(001) substrates coated with 100-nm thick SiO 2 . The film stack is composed of substrate/ d nm X/1 nm CoFeB/2 nm MgO|/1 Ta: the underlayer X is Hf, Ta, TaN and W. The TaN underlayer [37] is formed by reactively sputtering Ta in Ar gas atmosphere mixed with a small amount of N 2 . Ar and N 2 gas concentrations are controlled independently by gas mass flow meters. We define Q as the atomic ratio of the N 2 gas over the total (Ar+N 2 ) gas, that is, , where S X denotes the mass flow (in unit of sccm) of gas X. Q is varied from 0–2.5% here. The atomic composition of the TaN films is determined by Rutherford backscattering spectroscopy and the results are summarized in Supplementary Table 1 . All films are post annealed at 300 °C for 1 h in vacuum. Magnetic properties of the films are measured using vibrating sample magnetometry. The moment per unit volume ( M / V ) and the magnetic anisotropy energy ( K EFF ) are plotted in Supplementary Figs 6a–d, 7a–d, and 6e–h and 7e–h , respectively. To obtain M / V , saturated moment values ( M ) are divided by the product of film area and the nominal CoFeB thickness. It should be noted that the nominal thickness of the CoFeB layer contains, if any, the thickness of a magnetically dead layer. Thus M / V differs from the real saturation magnetization ( M S ) when a magnetic dead layer is present [37] . The magnetic anisotropy energy K EFF is estimated from the integrated difference of the out of plane and in-plane hysteresis loops. Positive K EFF corresponds to magnetic easy axis pointing along the film normal. Wires for evaluating current-induced domain wall motion and Hall bars for the analysis of current-induced effective field are patterned on the same wafer by optical lithography and Ar-ion etching. For these patterned films, the underlayer thickness ( d ) is varied within the substrate using a linear shutter during the sputtering. The underlayer thickness d of such ‘wedge film’ is calibrated by comparing the resistance of the patterned device (that is, a Hall bar) on the wedge film with that of a device patterned from a flat film in which the underlayer thickness is constant across the substrate. Wires used to study domain wall motion are ~5-μm wide and ~30-μm long (except one underlayer system X=TaN( Q :1.2%) for which we use ~15-μm long wires). The width w and length L of the Hall bars used here are ~10 μm and ~30–60 μm, respectively (see ref. 27 for the details). Subsequent lift-off process is used to make the 10 nm Ta/100 nm Au electrodes. Resistivity of each film is evaluated using the Hall bars. The underlayer thickness ( d ) dependence of the inverse of a normalized resistance (1/( R XX ˙ w / L )) is plotted in Supplementary Figs 6i–l and 7i–l for all underlayer films. Average resistivity values, obtained by the linear fitting shown in these figures, are tabulated in Supplementary Table 1 . For W, we find a jump in the resistivity at d ~5 nm (inset of Supplementary Fig. 6l ), suggesting that a structural phase transition (from β-W at small d to α-W at large d ) takes place at this thickness, as reported previously [31] . Note that the magnetic anisotropy K EFF of W/CoFeB/MgO heterostructures ( Supplementary Fig. 6h ) also drops as d exceeds ~5 nm. The y -axis intercept of the linear fitting of 1/( R XX ˙ w / L ) provides the resistivity of the CoFeB layer ( ρ CoFeB ). For the TaN underlayer films, which show a constant underlayer resistivity for a large d range, we find ρ CoFeB ~160 μΩ cm. Since it is difficult to estimate ρ CoFeB from the intercept for the other underlayer films, we assume ρ CoFeB ~160 μΩ cm throughout this paper. Separate CoFeB wedge films are made to check this assumption and we find relatively close values. Magneto-optical Kerr effect and the hysteresis loops Magneto-optical images of the wires are acquired using Kerr microscopy. To quantify the magnetic contrast, the region of interest (that is, the wire) is selected in the acquired image and converted into a two-dimensional arrays of integer. The average value of the Kerr intensity of the region of interest, denoted as I hereafter, is plotted in Supplementary Fig. 9a as a function of the out-of-plane field H z . Hysteresis loops of wires with different TaN( Q : 0.7%) underlayer thicknesses are shown. For the thicker underlayer films, I is larger when the magnetization is pointing up (large positive H z ). In contrast, I is larger for magnetization pointing downward for the thinner underlayer films. The difference in I when the magnetization is pointing ‘up’ and ‘down’ is defined as Δ I and the mean value of I is denoted as I 0 . Supplementary Fig. 9b shows Δ I / I 0 as a function of the underlayer thickness for three film structures. The sign of Δ I / I 0 changes at a certain thickness for each film structure. These changes in Δ I / I 0 are likely due to an optical interference effect within the sample including the 100-nm thick SiO 2 layer and the Si substrate. Note that we do not observe any change in the sign of Δ I / I 0 for the same film structure when we use naturally oxidized Si substrates. All images shown in this paper are subtracted images. An image of an uniformly magnetized state with magnetization pointing along – z is captured as the reference image. This reference image is subtracted from each image. Domain wall nucleation using current pulses A domain wall is nucleated by applying voltage pulses to the wire. First, the CoFeB layer is uniformly magnetized by applying an out-of-plane field H z . The field is then reduced to zero and we apply a voltage pulse (typically 100 ns of duration) to nucleate a domain wall. This process typically suffices to create one or two domain walls within the wire. In some film structures, an additional magnetic field application is required to change the domain pattern after the pulse application to form an appropriate domain structure. Propagation field of the domain walls The out-of-plane field needed to move a domain wall, that is, the propagation field H P , is evaluated using Kerr microscopy images. After the domain wall nucleation process, the out-of-plane field H z is ramped towards higher magnitude, either to positive or negative H z , and the magnetic state is monitored with the Kerr microscopy. Such measurement cycle is repeated in each device 10 times (five times for positive and five times for negative H z ). The propagation field H P is defined as the field ( H z ) at which the Kerr signal change exceeds 50% of the total change expected. The field ramp rate is approximately 1 Oe s −1 near the propagation field. Evaluation of current-driven domain wall velocity Current-induced domain wall motion is studied by applying voltage pulses to the wire, and the distance the domain wall travelled after the pulse application is evaluated using Kerr microscopy images. Typically, a pulse train consisting of 1–20 pulses (duration of each pulse is 20–100ns) separated by ~10 ms is applied to the sample and a Kerr image of the device is captured ~1 s after the pulse train application. This process is repeated multiple times to move a domain wall across the ~30-μm long wire. We fit the wall position as a function of cumulated pulse length with a linear function to obtain the wall velocity. In general, the velocity is nearly constant when the wall is moving. Once the wall gets pinned, the velocity is zero and these points are excluded from the fitting. Such processes of moving a domain wall across the wire are performed multiple times for a given pulse amplitude. Supplementary Fig. 10 shows exemplary profiles of how a domain wall propagates along the wire depending on the film structure. We find that the wall motion depends on the strength of spin Hall torque and/or spin transfer torque. If the size of spin Hall/spin transfer torque is strong enough, the wall moves along the wire relatively smoothly without pinning ( Supplementary Fig. 10a ). In contrast, when the spin Hall/spin transfer torque is small (for example, in TaN( Q : 2.5%) underlayer films), the domain wall often gets pinned at a local pinning center ( Supplementary Fig. 10b ). For such profiles, we fit the position versus cumulated pulse length only when the wall is moving and take an average value of the slopes. Current-induced effective field measurements Hall bars, patterned on the same wafer with the wires, are used to evaluate the current-induced effective field. The effective field is measured in the same manner as described in ref. 27 . A constant amplitude sinusoidal voltage (amplitude: V IN ) is applied to the Hall bar, and the in-phase first ( V ω ) and the 90° out-of-phase second ( V 2ω ) harmonic Hall voltages are measured using lock-in amplifiers. The resistance does not change with the voltage within the range we apply, thus the excitation can be treated as a constant amplitude sinusoidal current. An in-plane magnetic field directed along ( H L ) or transverse ( H T ) to the current flow is applied to evaluate the longitudinal ( ΔH L ) and transverse ( ΔH T ) components of the effective field, respectively. Contributions from the anomalous Hall effect and the planar Hall effect [28] are taken into account in obtaining ΔH L and ΔH T . The longitudinal and transverse components of the effective field are estimated using the following expressions [40] : where , and . Δ R P and Δ R A are the planar and anomalous Hall resistances, respectively. The plus/minus signs correspond to magnetization pointing along plus/minus z direction. The underlayer thickness dependences of Δ R A and Δ R P are shown in Supplementary Fig. 11a–f ; the ratio ξ of Δ R P to Δ R A is plotted in Supplementary Fig. 11g–l . Δ R A and Δ R P are obtained by measuring the change in the Hall resistance when the field is swept along the film normal or rotated within the film plane, respectively. The planar Hall effect is ~5% in magnitude of the anomalous Hall effect for the Hf, Ta and TaN underlayer films. For the W underlayer films, we find a large planar Hall effect contribution to the Hall resistance. This may be due to the interdiffusion of W with CoFeB, which may increase spin-dependent scattering within the CoFeB film. How to cite this article: Torrejon, J. et al . Interface control of the magnetic chirality in CoFeB/MgO heterostructures with heavy-metal underlayers. Nat. Commun. 5:4655 doi: 10.1038/ncomms5655 (2014).